Broadband light management using low-Q whispering gallery modes in spherical nanoshells Light trapping across a wide band of frequencies is important for applications such as solar cells and photodetectors. Here, we demonstrate a new approach to light management by forming whispering-gallery resonant modes inside a spherical nanoshell structure. The geometry of the structure gives rise to a low quality-factor, facilitating the coupling of light into the resonant modes and substantial enhancement of the light path in the active material, thus dramatically improving absorption. Using nanocrystalline silicon (nc-Si) as a model system, we observe broadband absorption enhancement across a large range of incident angles. The absorption of a single layer of 50-nm-thick spherical nanoshells is equivalent to a 1-μm-thick planar nc-Si film. This light-trapping structure could enable the manufacturing of high-throughput ultra-thin film absorbers in a variety of material systems that demand shorter deposition time, less material usage and transferability to flexible substrates. Broadband light management is an essential design consideration for high-performance solar cells, as well as other optical devices such as photodetectors. For example, surface texturing [1] and reflectors [2] are used to improve the in-coupling of light and enhance optical path length in many types of conventional thick- and thin-film solar cells [3] . When the structure size is comparable to or even smaller than the wavelength, two main light-trapping approaches, photonic crystals [4] , [5] and plasmonic nanostructures [6] , [7] , [8] have been extensively studied. A photonic crystal can be used either as an omnidirectional lossless reflector [4] or a diffractive element outside the photoactive layer [5] , [9] , or as a photoactive absorber [10] , [11] , [12] , [13] , [14] , [15] , [16] , [17] to couple incident light into quasi-guided modes. Plasmonic nanostructures enhance light absorption because they can scatter incident light into wave-guided modes [18] or surface plasmon-polariton modes [19] , [20] , or increase the optical electric field around nanostructures [21] . Whispering gallery mode (WGM) resonators operating at optical frequencies have been successfully used to build laser cavities, filters, sensors and wave mixers [22] , [23] , [24] , [25] . In these applications, resonators with a quality factor (Q) ranging from 10 5 to 10 9 or even higher are preferred, because high-Q resonators have very little energy leakage and high-frequency selectivity at the expense of a low coupling efficiency of light into the resonator. In contrast, the application of WGMs to broadband absorbers requires the opposite resonator characteristics, such as high absorption, low frequency selectivity and strong in-coupling, which favor low-Q. However, very few applications based on low-Q WGM resonators have been explored so far. In this work, we take advantage of low-Q WGMs in spherical nanoshells to dramatically enhance broadband absorption. Most of the incoming light couples into the WGMs in the spherical nanoshells and circulates in the active material with a considerably longer path length than the same material in the form of planar film, thereby substantially reducing the amount of material required for sufficient light absorption. We choose nanocrystalline silicon (nc-Si) to demonstrate this concept. nc-Si consists of 1–50 nm small crystalline grains embedded in amorphous Si (a-Si) matrix [26] , [27] . It is an important photovoltaic material due to its 1.1 eV band gap and high robustness to light-induced degradation compared with a-Si, and its higher 'apparent' absorption coefficient compared with mono-crystalline silicon [27] . nc-Si cells are used in tandem with a-Si cells in industry (micromorph solar cells); such micromorph cells have an 11.9% champion efficiency [28] . An important constraint on manufacturing the nc-Si cells is the need for thick (~2 μm) films due to the low-absorption coefficient. Achieving thick, high-quality nc-Si films at fast deposition rates has proven to be challenging [29] . Under standard plasma-enhanced chemical vapor deposition (13.56 MHz frequency) conditions, where the deposition rate is ~1 Å s −1 , it takes more than 5 h to deposit a 2-μm-thick film, which is too long considering the high throughputs needed for solar-cell production and leads to a high device cost [30] . Hence, reducing the cell thickness by taking advantage of light trapping is very attractive for nc-Si. Random-textured transparent conductive electrodes, such as boron-doped ZnO by low-pressure chemical vapor deposition (LPCVD) [31] , [32] , are currently used at an industrial scale for light trapping in such devices. We demonstrate that a nanoshell semiconductor absorber less than 100nm thick can achieve performance similar to a micron-thick planar geometry, thereby reducing the film deposition time from hours to minutes; this thickness of absorber is comparable to the thickness of organic absorbers, but has heretofore not been possible in inorganic solar cell systems. The application of WGM-enhanced absorption for wide-band light management opens the door to various solar cell, solar fuel and photodetector applications. Enhanced absorption in nc-Si spherical nanoshells The preparation of spherical nanoshells is quite simple and scalable. First, monodispersed suspensions of colloidal silica nanospheres were prepared following the modified Stöber method [33] ; these spheres were then coated onto 4-inch quartz-wafer substrates using the Langmuir–Blodgett (LB) method. The LB approach can be repeated for multi layers and could also be replaced by any large-scale technique suitable for depositing monolayers of particles, for example, the rod-coating technique developed in our group [34] . Next, nc-Si was conformally deposited on the surface of the silica spheres by LPCVD of SiH 4 at 620 °C, with a rate of 10 nm min −1 . Finally, the silica cores were removed by dipping the samples in a 5% dilute hydrofluoric acid solution. The method is similar to the intercalation of self-assembled synthetic opals described by Vlasov et al . [35] . Instead of focusing on the photonic band structure of the ordered sphere array [35] , we are exploring light trapping due to whispering gallery resonances within the nanoshells. 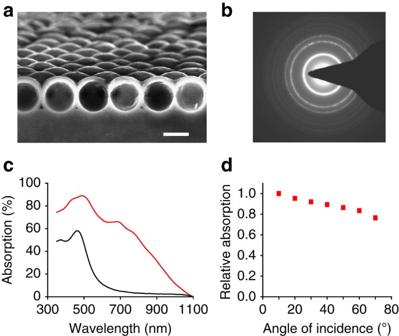Figure 1: Nanocrystalline Si spherical nanoshell morphology and optical absorption. (a) SEM cross-sectional image of a monolayer of Si spherical nanoshells on a quartz substrate. Scale bar equals 300 nm. (b) Electron diffraction pattern showing the nanocrystalline nature of Si. (c) Integrating sphere measurement of absorption spectra under normal incidence for the flat sample (black line) and nanoshell sample (red line). (d) Integrated absorption over the global solar spectrum (ASTM G173-03) for different incidence angles relative to normal incidence. Figure 1a shows the cross-sectional scanning electron microscope (SEM) image of a monolayer of spherical nanoshells on a quartz substrate. The electron diffraction pattern obtained by transmission electron microscope ( Fig. 1b ) confirms the nanocrystalline nature of the sample. The Si deposition thickness is 50 nm, and a flat sample was deposited side-by-side as a control. We measured the absorption of both samples using an integrating sphere. Figure 1c shows that the spherical nanoshells absorb significantly more than the flat sample over a broad region, particularly in the near-infrared range where nc-Si absorbs weakly. To estimate the optical path length, a wavelength of 700 nm is selected as an example where the absorption coefficient for nc-Si is 4×10 3 cm −1 (ref. 27 ). The optical path length for the flat sample is calculated to be ~50 nm (Methods), whereas the optical path for spherical nanoshells sample is 1,000 nm, suggesting an optical path enhancement factor of 20. The spherical nanoshell monolayer can absorb 60% of the above-bandgap solar spectrum as compared with the flat sample's 18%. The absorption enhancement is also relatively insensitive to angle of incidence, particularly in the near-infrared regime; as shown in Figure 1d , integrated absorption shows a maximum variation of less than 25% between normal incidence and incidence at 70° from the normal. Figure 1: Nanocrystalline Si spherical nanoshell morphology and optical absorption. ( a ) SEM cross-sectional image of a monolayer of Si spherical nanoshells on a quartz substrate. Scale bar equals 300 nm. ( b ) Electron diffraction pattern showing the nanocrystalline nature of Si. ( c ) Integrating sphere measurement of absorption spectra under normal incidence for the flat sample (black line) and nanoshell sample (red line). ( d ) Integrated absorption over the global solar spectrum (ASTM G173-03) for different incidence angles relative to normal incidence. Full size image Elucidation of the low-Q WGM mechanism Light scattering by a dielectric concentric spherical shell has been studied previously and can be formally solved [36] , [37] . To better understand the light-trapping effect, we performed full-wave simulations for the nanoshell structures. 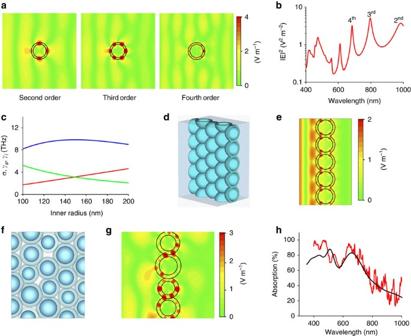Figure 2: Optical simulations of Si spherical nanoshells. (a) Electric field (|E|) distribution based on full-wave simulations of electromagnetic waves coupled with a single Si nanoshell (inner radiusRin=175 nm, outer radiusRout=225 nm). Resonance wavelengths are 986, 796 and 685 nm, respectively. Light is incident from left-hand side with an amplitude of 1 V m−1for all wavelengths with the electric field perpendicular to the paper plane. (b) |E|2versus wavelength at the right-most point of the nanoshell showing resonant peaks corresponding to resonance modes in panel (a). (c) Spectral cross-section σ (blue), external leakage rateγe(red) and intrinisic loss rateγi(green), as a function of the inner radius for the third order resonance, where the thickness of the spherical shell is fixed as 50 nm. (d) Schematic of a hexagonal array of nanoshells (Rin=175 nm,Rout=225 nm) based on which full-wave simulations were performed. (e) Electric-field (|E|) distribution in the model in panel (d) at 594 nm. SeeSupplementary Movie 1for an animated version of this image. (f) Front view of a spherical nanoshell array with variations in geometry. (Rin=175±25 nm, shell thicknessRshell=80±5 nm). (g) Side view of the electric-field (|E|) distribution in the model in panel (f) at 860 nm. The smallest nanoshell shows a field distribution close to resonance, whereas the largest nanoshell is off-resonance. (h) Experimentally measured absorption spectrum (black) of LPCVD deposited nc-Si nanoshell sample (Rin~175 nm, Rshell~80 nm) and simulated absorption spectrum (red) based on full-wave simulations of the structure in panel (f). Figure 2a shows the amplitude of the WGM electric-field patterns at 986, 796 and 685 nm, respectively, corresponding to the second-, third- and fourth-order resonances of a single spherical nanoshell ( R in =175 nm and R out =225 nm). Incident plane waves come from the left side with the electric field perpendicular to the paper plane and with an amplitude of 1 V m −1 . Light is confined and guided along the shell instead of directly passing through the shell. The round shape of the shell forms a closed path for light and causes resonance at certain frequencies. The circulation of electromagnetic waves inside the nanoshell leads to the accumulation of electromagnetic energy inside the active material (nc-Si). Figure 2b plots the light intensity versus wavelength at the right-most point of the spherical nanoshell. The low-order resonances show broadband enhancements and contribute to the significant enhancement in the long wavelength regime. The absorption peaks are further broadened due to variations in their spherical geometry, which will be discussed in more detail at the end of this section. Figure 2: Optical simulations of Si spherical nanoshells. ( a ) Electric field (|E|) distribution based on full-wave simulations of electromagnetic waves coupled with a single Si nanoshell (inner radius R in =175 nm, outer radius R out =225 nm). Resonance wavelengths are 986, 796 and 685 nm, respectively. Light is incident from left-hand side with an amplitude of 1 V m −1 for all wavelengths with the electric field perpendicular to the paper plane. ( b ) |E| 2 versus wavelength at the right-most point of the nanoshell showing resonant peaks corresponding to resonance modes in panel ( a ). ( c ) Spectral cross-section σ (blue), external leakage rate γ e (red) and intrinisic loss rate γ i (green), as a function of the inner radius for the third order resonance, where the thickness of the spherical shell is fixed as 50 nm. ( d ) Schematic of a hexagonal array of nanoshells ( R in =175 nm, R out =225 nm) based on which full-wave simulations were performed. ( e ) Electric-field (|E|) distribution in the model in panel ( d ) at 594 nm. See Supplementary Movie 1 for an animated version of this image. ( f ) Front view of a spherical nanoshell array with variations in geometry. ( R in =175±25 nm, shell thickness R shell =80±5 nm). ( g ) Side view of the electric-field (|E|) distribution in the model in panel ( f ) at 860 nm. The smallest nanoshell shows a field distribution close to resonance, whereas the largest nanoshell is off-resonance. ( h ) Experimentally measured absorption spectrum (black) of LPCVD deposited nc-Si nanoshell sample ( R in ~175 nm, R shell ~80 nm) and simulated absorption spectrum (red) based on full-wave simulations of the structure in panel ( f ). Full size image The resonant modes in the shells enhance light trapping and absorption, whereas their relatively low-Q not only enable good coupling between propagating light and resonant modes, but also broaden the resonant absorption peak and make the absorption enhancement region wider. To optimize the light-trapping capability for a single resonance, it is necessary to optimize the spectral cross-section , where γ e and γ i correspond to the external leakage rate and the intrinsic loss rate, respectively [9] . The spectral cross-section is the integration of the absorption coefficients over the spectrum of the resonance lineshape and it measures the contribution of a single resonance to broadband light-trapping absorption enhancement. For our spherical nanoshell structure, we use the Mie theory [38] to calculate the resonant frequency, γ e and γ i . When the thickness of the spherical shell is fixed at 50 nm, the variations of the spectral cross-section σ, as well as γ e and γ i , as a function of the inner radius d are plotted in Figure 2c . We have chosen to examine the third resonance, because its resonant wavelength is located in the long wavelength range where light trapping should be the most beneficial. The spectral cross-section features a maximum around d ~150 nm. Such a maximum results from competition between two trends. The enhancement factor over a single pass optimizes at the limit of γ e ≫ γ i (ref. 9 ), which favors a thicker d . On the other hand, γ i decreases with a thicker d . We note that the maximum is fairly broad in d , indicating a basic robustness in terms of light-trapping capability in this structure. This simulation result is the guideline for our experimental sphere-size choice, and our sample with optimized sizes ( R in =175 nm) in Figure 1 has shown very effective absorption enhancement. Our calculation shows that the Q factors, where both the external leakage and the intrinsic loss are considered in the resonant dissipation, range from 20 to 100 for the second and third modes. On the basis of the definition of Q, one can easily estimate that light can circulate around the circumference of the shell for one to three rounds before its energy is reduced to 1/e. In other words, the light path has been increased by a few tens of times, which is consistent with our experimental observations in Figure 1c . Figure 2d shows the schematic of a spherical shell array whose electrical field pattern in the cross section along one of the shell rows is given in Figure 2e . Supplementary Movie 1 vividly shows that light (594 nm) is guided inside the shell array. We see very strong resonant enhancement even when the shells are touching each other. Although close packing induced some cross talk between neighboring nanoshells, it did not harm the effect of light trapping as shown by our simulation results. In a large ensemble of nanoshells, variation in their geometry can further broaden the absorption peaks. To simulate this effect, we created a spherical nanoshell array structure ( Fig. 2f ) with varying sphere size ( R in =175±25 nm) and shell thickness ( R shell =80±5 nm) supported by SEM images of our sample. Figure 2g shows the electric-field distribution inside the modified nanoshell array at 860 nm. WGMs are formed in the nanoshells. We can see that the smallest nanoshell is close to the resonance condition, whereas the biggest nanoshell is off-resonance, which clearly demonstrates that the geometry variation leads to a broad distribution of resonant wavelengths. The simulated absorption spectrum ( Fig. 2h ) shows the smearing of the resonant peaks and in good agreement with the experimental curve. Effect of nanoshell thickness To further elucidate the optical properties of spherical nanoshells, we studied the effect of shell thickness on optical absorption. 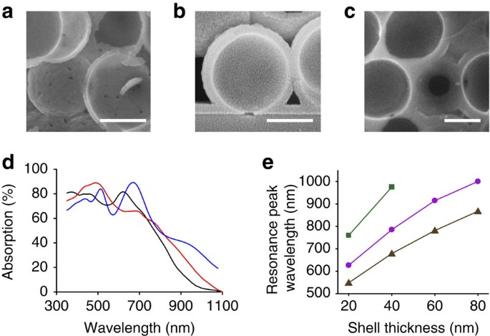Figure 3: Effect of shell thickness on the optical properties of nc-Si spherical nanoshells. (a–c) Cross-sectional SEM images of nc-Si spherical nanoshells with Si deposition time of 2.5, 5 and 12 min, respectively. Scale bar equals 200 nm. (d) Absorption spectra for spherical nanoshells with Si deposition times of 2.5 (black), 5 (red) and 12 (blue) min, respectively. (e) Full-wave simulation results of peak wavelength of 2nd (dark green), 3rd (purple) and 4th (brown) order resonance versus shell thickness for a single spherical nanoshell withRin=200 nm. Figure 3 shows the effect of shell thickness on the absorption spectrum, Figure 3a–c show cross-sectional SEM images for nc-Si shells deposited in LPCVD for different periods of time. The shell thicknesses are 25 and 50 nm for 2.5 and 5 min depositions, respectively. When the deposition time increases to 12 min, Si fills in the void space of the packed silica nanospheres and forms the inverse opal structure. Figure 3d compares the absorption spectrum for these samples, and the absorption peaks are found to red-shift with increasing shell thickness. To understand this red-shift phenomenon, we modeled the shift of second, third and fourth resonance peaks with increasing shell thickness in Figure 3e . Similar to traditional planar waveguides, when the shell thickness gets thicker, the transverse components of the wavevector become smaller, whereas the longitudinal components become larger, which means that the effective wavelength along the shell becomes shorter. Therefore, the resonant frequency for the modes with the same number of lobes shows a red-shift behavior, in agreement with our experimental data ( Fig. 3d ). This further confirms that the WGM resonances are fundamental to absorption enhancement in the spherical nanoshell structure. Figure 3: Effect of shell thickness on the optical properties of nc-Si spherical nanoshells. ( a – c ) Cross-sectional SEM images of nc-Si spherical nanoshells with Si deposition time of 2.5, 5 and 12 min, respectively. Scale bar equals 200 nm. ( d ) Absorption spectra for spherical nanoshells with Si deposition times of 2.5 (black), 5 (red) and 12 (blue) min, respectively. ( e ) Full-wave simulation results of peak wavelength of 2nd (dark green), 3rd (purple) and 4th (brown) order resonance versus shell thickness for a single spherical nanoshell with R in =200 nm. Full size image Effect of number of nanoshell layers To further demonstrate the potential for nanoshells in ultra-thin solar cell architectures, we constructed nanoshell arrays with multiple layers through sequential LB coatings before nc-Si deposition. 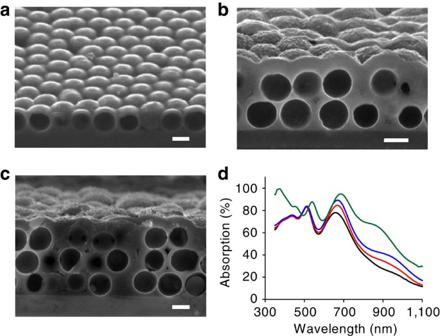Figure 4: Effect of number of nanoshell layers on optical properties. (a–c) Cross-sectional SEM images of one to three layers of spherical nanoshells. Scale bar equals 300 nm. (d) Absorption spectra corresponding to different numbers of layers of spherical nanoshells: one layer (black), two layers (red), three layers (blue). A 100-nm thick tin-doped indium oxide (ITO) AR layer coating (dark green) further improves absorption of the three-layer film, with a total absorption of 75% of the above-bandgap solar spectrum. Figure 4 shows the cross-sectional SEM images of one, two and three layers of nanoshells, and the absorption spectrum of each sample. We observed two regimes in the absorption spectrum. For the short wavelength region (<500 nm), increasing the number of layers does not increase the absorption ( Fig. 4d ). This is because the absorption coefficient of nc-Si in this region is high (>1×10 5 cm −1 ) [39] ; therefore, all of the light loss can be attributed to light reflection. As the top surfaces of samples with different numbers of layers ( Fig. 4a–c ) have a similar shape, the anti-reflection (AR) effect would be expected to be similar, resulting in no change in absorption. For wavelengths above 500 nm, we observed increased absorption with the number of layers. For example, at 900 nm, the absorption increases from 27% for one layer to 34% for two layers, and to 41% for three layers. The integrated absorption increases by 6% between the single- and triple-layer samples. Further coating of the three-layer structure with an AR coating (100-nm thick, tin-doped indium oxide) improves near-infrared absorption, with a total absorption of 75% of the above-bandgap solar spectrum. This shows that a single layer is more cost effective in absorbing a significant portion of incoming light, yet the performance of the structure can be further improved in circumstances where high absorption is more important. The obviation of the need for thicker films or additional layers is particularly important for solar cells constructed from rare absorber materials such as cadmium telluride or copper indium gallium selenide. The impact of our light-trapping structure is therefore relevant to the economics of devices in various material systems. Figure 4: Effect of number of nanoshell layers on optical properties. ( a – c ) Cross-sectional SEM images of one to three layers of spherical nanoshells. Scale bar equals 300 nm. ( d ) Absorption spectra corresponding to different numbers of layers of spherical nanoshells: one layer (black), two layers (red), three layers (blue). A 100-nm thick tin-doped indium oxide (ITO) AR layer coating (dark green) further improves absorption of the three-layer film, with a total absorption of 75% of the above-bandgap solar spectrum. Full size image Transferability to a flexible substrate Moreover, nanoshells are amenable not only to multiple material systems, but also to multiple substrates. For example, the spheres can be lifted off the quartz substrate by etching and transferred onto flexible substrates, such as polydimethylsiloxane. 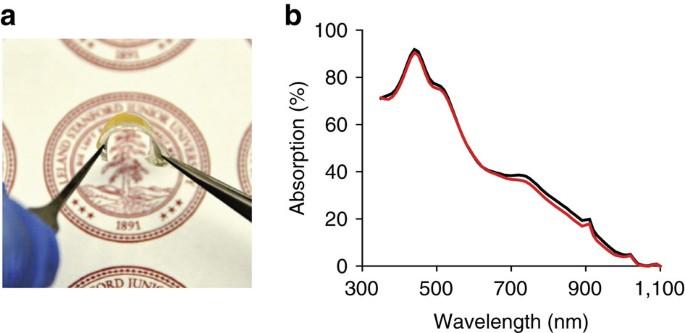Figure 5: Transferability of spherical nanoshells to a flexible substrate. (a) A photo of nc-Si spherical nanoshells transferred to a polydimethylsiloxane (PDMS) substrate and bent at a radius of 8 mm. (b) Absorption spectrum of nc-Si spherical nanoshells on PDMS substrate when laying flat (black line) and bent at a radius of 8 mm (red line). Figure 5a shows a photo of a single layer of nc-Si spherical nanoshells on a polydimethylsiloxane substrate and bent at a radius of 8 mm. Figure 5b shows little change in the absorption curve when the sample is lying flat or bent at a radius of 8 mm, indicating the robustness of WGM-based light trapping. Facile transfer coupled with low angle dependence of absorption suggests that spherical nanoshells on a flexible substrate could be bent according to the shape of the underlying object. Figure 5: Transferability of spherical nanoshells to a flexible substrate. ( a ) A photo of nc-Si spherical nanoshells transferred to a polydimethylsiloxane (PDMS) substrate and bent at a radius of 8 mm. ( b ) Absorption spectrum of nc-Si spherical nanoshells on PDMS substrate when laying flat (black line) and bent at a radius of 8 mm (red line). Full size image Electrical simulation Finally, we conducted a theoretical simulation on the performance of a p-i-n solar cell, based on the spherical nanoshell array structure. 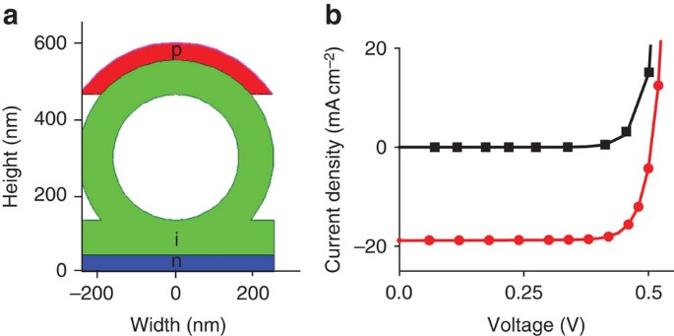Figure 6: Theoretical study of electrical performance of a p-i-n solar cell structure. (a) p-i-n structure with a 40-nm thick top p layer (red) with doping concentration 1×1018cm−3, i (intrinsic, green) spherical nanoshell layer with inner radius 145 nm and outer radius 225 nm, and bottom 40-nm-thick n layer (blue) with doping concentration 1×1018cm−3. (b) Simulated J-V curve under illumination (red) and in the dark (black). Figure 6a shows the cross-section of one sphere in the array. In this structure, a single layer of undoped hollow Si spheres with a thickness of 80 nm and an outer radius of 225 nm sits atop a 40-nm thick, n-type (1×10 18 cm −3 ) substrate. A 40-nm p-type (1×10 18 cm −3 ) layer caps the spheres. We approximated the optical generation of electrons as a constant profile by assuming that 75% of the above-bandgap photons are absorbed. Radiative, Shockley–Read–Hall, and Auger recombination in the semiconductor layers and surface recombination at the semiconductor interfaces were accounted for in the simulation, using standard coefficients for silicon. From the simulated J-V curve ( Fig. 6b ), V oc =0.51 V, J sc =20.1 mA cm −2 , FF=79.0% and η =8.1%. To achieve similar short-circuit current density and efficiency using a flat nc-Si cell would require an active layer thickness of approximately 1.5 μm [40] . In addition to the high short-circuit current afforded through enhanced absorption, the open-circuit voltage of the nanoshell solar cell is comparable to that of a planar design (0.51 versus 0.54 V (ref. 40 )), indicating that the interfacial recombination due to increased surface area is well controlled in the p-i-n architecture. There are many challenges to be overcome to maintain high open-circuit voltage in nanoshell solar cells in practice, including film quality and uniformity, surface passivation, and the development of growth conditions that promote good interfaces and avoid significant dopant diffusion. However, simulations show that if these challenges are addressed, solar cells using the WGM light-trapping scheme fundamentally have the potential to achieve excellent performance with reduced material use and improved manufacturing throughput. Figure 6: Theoretical study of electrical performance of a p-i-n solar cell structure. ( a ) p-i-n structure with a 40-nm thick top p layer (red) with doping concentration 1×10 18 cm −3 , i (intrinsic, green) spherical nanoshell layer with inner radius 145 nm and outer radius 225 nm, and bottom 40-nm-thick n layer (blue) with doping concentration 1×10 18 cm −3 . ( b ) Simulated J-V curve under illumination (red) and in the dark (black). Full size image Using spherical nanoshell structures, we achieved absorption comparable to micron-thick layers with 50-nm-thick shells, reducing the film deposition time necessary to achieve strong absorption from hours to minutes. Macroscale spherical silicon solar cells have been previously demonstrated by Texas Instruments with spheres of ~0.4 mm in size [41] . We have shown that when the size of sphere is reduced to the optical wavelength scale, new optical phenomena can be exploited for broadband light absorption. The mechanism of light management in spherical nanoshells is substantially different from using particles as scattering centers to increase path length [42] , [43] . The Si nanoshells show good confinement in WGM due to the high-index contrast between the air/substrate and the nc-Si ( n =3.5) while maintaining low-Q to facilitate in-coupling. The optical response of the nanoshells can also be tuned by changing the waveguide properties, such as the thickness. We also showed the versatility of the technique, demonstrating further enhancement of absorption through the use of multiple layers and an AR coating for applications where absorption is critical, transferring the nanoshells to a flexible substrate and simulating a potential solar cell structure. Silica nanosphere synthesis and assembly Silica nanospheres were synthesized following the modified Stöber synthesis [33] . While stirring the tetraethyl orthosilicate solution with ethanol, NH 4 OH mixed with ethanol was added. The solution was cleaned with ethanol and methanol after 4 h of reaction, producing silica nanospheres. Silica nanospheres were then modified with aminopropyl methyldiethoxysilane, so that they could be terminated with positively charged amine groups to prevent aggregation. These modified nanospheres were then injected into an LB trough (KSV 5000) using a syringe pump. Finally, they were assembled into closed-packed layers on 4-inch quartz wafer substrates via the LB method. By repeating dipping and drying multiple times, this method can be used to create multiple layers of closed-packed silica layers. nc-Si spherical nanoshells fabrication Quartz wafers coated with silica nanospheres were loaded into the LPCVD tube furnace at the Stanford Nanofabricaiton Facility. Si was deposited onto the surface of silica at a low pressure (~500 mtorr) using silane (SiH 4 ) at 620 °C. The deposition rate at this temperature is ~10 nm min −1 . When the target silicon thickness was reached, the sample was taken out of the furnace. The silica cores were removed by dilute hydrofluoric acid etching for 5 min. Optical measurements Standard hemispherical measurements were carried out with an integrating sphere (Newport). A xenon lamp coupled to a monochromator was used for both wavelength-dependent and incident-angle-dependent measurements. The sample was mounted at the centre of the sphere. The reflected light and transmitted light from the sample were uniformly scattered by the integrating sphere and collected by a photodetector. In this study, all light reflected from and transmitted through the sample was accounted for, so this can be considered a measurement of the absolute absorption. Estimation of optical path lengths The optical path length is estimated according to Beer's law [44] , which states that there is a logarithmic dependence between the transmission ( T ) of light through a substance and the product of the absorption coefficient of the substance (α) and the distance the light travels through the material (that is, the path length, ℓ ): . So the optical path length can be calculated as where A is the measured absorption and α of nc-Si at 700 nm is 4×10 3 cm −1 (ref. 27 ). Optical simulation The optical simulations were conducted using the commercial software package CST Microwave Studio. The full-wave calculation is based on a finite integration technique, which uses the integral form of the Maxwell equations as compared to the finite-difference time-domain methods. The response of the shells was analyzed using linearly polarized plane-wave excitation. Electrical simulation The electrical simulation of the spherical nanoshell p-i-n solar cell structure was conducted using Synopsis Sentaurus, which solves the Poisson and continuity equations over a mesh of the structure (with periodic boundary conditions assumed in the plane of the spheres). The optical-generation profile was assumed to be constant through the entire structure based on 75% absorption of photons, and the electrical material properties were taken as the default values for crystalline silicon as stored in the Sentaurus material database. Shockley–Read–Hall, Auger and surface recombination in the semiconductors were taken into account, using the models for crystalline Si in Sentaurus. Recombination at the contacts and contact resistance were not included in this simulation. How to cite this article: Yao, Y. et al . Broadband light management using low-Q whispering gallery modes in spherical nanoshells. Nat. Commun. 3:664 doi: 10.1038/ncomms1664 (2012).